The yeast regulator of transcription protein Rtr1 lacks an active site and phosphatase activity The activity of RNA polymerase II (Pol II) is controlled in part by the phosphorylation state of the C-terminal domain (CTD) of its largest subunit. Recent reports have suggested that yeast regulator of transcription protein, Rtr1, and its human homologue RPAP2, possess Pol II CTD Ser5 phosphatase activity. Here we report the crystal structure of Kluyveromyces lactis Rtr1, which reveals a new type of zinc finger protein and does not have any close structural homologues. Importantly, the structure does not show evidence of an active site, and extensive experiments to demonstrate its CTD phosphatase activity have been unsuccessful, suggesting that Rtr1 has a non-catalytic role in CTD dephosphorylation. The activity of RNA polymeraes II (Pol II) is regulated by the phosphorylation state of the C-terminal domain (CTD) of its largest subunit [1] , [2] , [3] , [4] , [5] , which contains the consensus heptapeptide repeat Tyr1-Ser2-Pro3-Thr4-Ser5-Pro6-Ser7 (YSPTSPS). While all the hydroxyl groups in this repeat can become phosphorylated, phosphorylation of Ser2 and Ser5 has received the most attention to date. For example, phosphorylated Ser5 (pSer5) is found at the promoter and during the initiation and early stages of Pol II transcription, and it mediates the recruitment of the 5′-end capping machinery and other factors. pSer5 is then dephosphorylated, and Ser2 becomes phosphorylated during the elongation and termination stages of transcription, which also facilitates 3′-end processing of the pre-mRNA transcript. In keeping with the importance of Ser2 and Ser5 phosphorylation, the kinases and phosphatases involved have been well studied [5] . The phosphatase Fcp1 is present along the length of transcribed genes, and can dephosphorylate both pSer2 and pSer5, but prefers pSer2 [6] , [7] . Ssu72 is a known CTD pSer5 phosphatase [8] , [9] , although it is localized primarily near the 3′-end of genes. Ssu72 prefers the cis configuration of the pSer5-Pro6 peptide bond [10] , [11] , and it helps to couple transcription and polyadenylation [10] . Scp1 is another pSer5 phosphatase in metazoans, and it may function near the 5′ end of certain genes [12] , [13] , [14] . It was recently reported that the yeast protein Rtr1 ( r egulator of tr anscription [15] ) has Pol II CTD pSer5 phosphatase activity and is required for pSer5 dephosphorylation in the early stage of transcription [16] . The human homologue of Rtr1, RPAP2 (RNA Pol II-associated protein 2 [17] ), has also been reported to have CTD pSer5 phosphatase activity [18] . These proteins are poorly conserved overall ( Fig. 1 ), but they share a motif with three strictly conserved Cys residues and another residue conserved as His (in most fungi) or Cys (in animals and S. pombe , Fig. 1 ), suggestive of a zinc finger motif [15] . However, the spacing among these residues (C-X 4 -C-X n -C-X 3 -H/C, where n ranges from 30 to 50) as well as the sequences of Rtr1 homologues are distinct from known zinc finger proteins. Figure 1: Sequence conservation among Rtr1 and RPAP2 homologues. Sequence alignment of full-length K. lactis , S. cerevisiae and A. gossypii Rtr1 (KlRtr1, ScRtr1, AgRtr1) and human RPAP2 (HsRPAP2, residues 1–240 only, out of 612 residues total) is shown. The four zinc ligand residues are shown in orange. Residues conserved among 11 fungal Rtr1 homologues (excluding the second Rtr1 homolog in S. cerevisiae ) or 8 animal RPAP2 homologues are shown in magenta. Residues conserved among fungal Rtr1 and animal RPAP2 homologues are shown in blue. Residues not observed in the crystal structure of KlRtr1 are shown in lower-case italic. The secondary structure elements (S.S.) are labelled. Full size image In this study, we report the crystal structure of Rtr1. It reveals a new type of zinc finger protein, in fact distinct from other known protein structures in general. However, the structure lacks an apparent active site, and the zinc ion probably has a structural role, likely stabilizing the overall structure of the protein. Moreover, extensive efforts to demonstrate CTD phosphatase activity for Rtr1 from several different fungal species as well as for human RPAP2 were unsuccessful, in contrast to the earlier reports but consistent with the structural observations. Therefore, Rtr1/RPAP2 itself is unlikely a phosphatase, but perhaps has a non-catalytic role in CTD dephosphorylation. The identity of the pSer5 phosphatase in the early stage of Pol II transcription remains to be determined. Overall structure of Rtr1 We have determined the crystal structure of Kluyveromyces lactis Rtr1 (KlRtr1) at 2.5 Å resolution ( Table 1 , Supplementary Fig. S1 ). The bacterial growth media was supplemented with zinc during protein expression, and the purified protein had nearly stoichiometric amounts of zinc [19] . Fluorescence scans were carried out on the crystal at the absorption edges of Zn, Ni, Co and Fe, and anomalous signals were observed only at the Zn edge, which were used to solve the structure. The full-length protein (residues 1–211) was used for crystallization, but only residues 1–152 were observed in the structure. SDS gels of the crystals showed that the C-terminal segment of KlRtr1 was removed by proteolysis during crystallization ( Supplementary Fig. S2 ). The sequence conservation for these C-terminal residues is much weaker among Rtr1 and RPAP2 homologues ( Fig. 1 ). Table 1 Summary of crystallographic information. Full size table The structure of KlRtr1 (residues 1–152) contains five anti-parallel α-helices (αA–αE, Fig. 2a ). A long loop (residues 70–112) connects helices αD and αE, and the three strictly conserved Cys residues (73, 78 and 111) are located in this loop. Residues 88–100 at the tip of this loop are disordered in the current structure ( Fig. 2a ), and this loop may have also been proteolysed in some of the Rtr1 molecules in the crystal ( Supplementary Fig. S2 ). The fourth ligand to the zinc ion, His115 or Cys, is in the first turn of helix αE. This helix is followed by another long loop (residues 126–152) that wraps around one side of the structure ( Fig. 2a ). Figure 2: Rtr1 is a new type of zinc finger protein. ( a ) Schematic drawing of the structure of K. lactis Rtr1. The zinc atom is shown as a sphere (in orange), and its four ligands are shown as stick models (in cyan). The two views are related by a rotation of ~60° around the vertical axis. ( b ) Simulated annealing omit F o –F c electron density for the zinc atom and its ligands in the structure of KlRtr1 at 2.5 Å resolution, contoured at 2.5σ. ( c ) Overlay of the zinc-binding site of K. lactis Rtr1 (in colour) and the zinc finger domain of Rabex-5 (in grey). The superposition is based on the first two zinc ligands. All the structure figures were produced with PyMOL ( www.pymol.org ). Full size image We also obtained crystals of Ashbya gossypii Rtr1 (AgRtr1), although the best diffraction data set extended only to 3.5 Å resolution. By combining the structural information from KlRtr1 and primary phase information from Zn anomalous signals, we were able to observe another helix in the C-terminal region of AgRtr1, likely equivalent to residues 154–166 of KlRtr1 ( Fig. 1 ). This helix is projected away from the rest of the protein and is stabilized by crystal packing interactions in the AgRtr1 crystal ( Supplementary Fig. S3 ), suggesting that the C-terminal region of Rtr1 may function independently of the N-terminal region. Rtr1 is a new type of zinc finger protein The zinc ion is coordinated in a tetrahedral fashion by the four conserved ligands ( Fig. 2a and b ). The zinc-binding site is located near the surface, but there are no prominent features in this region of the protein (see below). The main-chain carbonyl oxygen atoms of the first two ligands, Cys73 and Cys78, are hydrogen bonded to the guanidinium group of Arg67, one of the few other conserved residues among these proteins ( Fig. 1 ). The hydrogen bonds stabilize the two Cys residues as well as the loop connecting them, which is hydrophobic in nature and contributes to the formation of the hydrophobic core of Rtr1 ( Fig. 2a ). The zinc ion therefore seems to have a structural role, likely stabilizing the overall conformation of Rtr1. We have identified Rtr1 as a new type of zinc finger protein. A search through the Protein Data Bank with DaliLite [20] did not identify any close structural homologues, with the highest Z score being 3.3. The overall fold of Rtr1 is somewhat reminiscent of the HEAT repeats, although the positions of the helices are different compared with these repeats. The topology of the zinc ligands in Rtr1, with the first three located in loops and the last one in the beginning of a helix, has some similarity to the A20 family of zinc finger proteins [21] , as illustrated by the structure of Rabex-5, a guanine nucleotide exchange factor for Rab5 that also binds monoubiquitin [22] , [23] . The overall conformations of the protein backbone near the first two zinc ligands are similar between Rtr1 and Rabex-5 ( Fig. 2c ). On the other hand, the loop connecting them, and especially the loop connecting to the third ligand, has different numbers of residues (the zinc ligands in Rabex-5 have the motif C-X 3 -C-X 11 -C-X 2 -C). In addition, the orientation of the helix containing the fourth ligand differs by nearly 90° between the two structures. Finally, the zinc-binding site in Rtr1 is part of a much larger structure, with 150 residues ( Fig. 2a ), whereas the zinc finger domain of Rabex-5 contains only 35 residues. Purified Rtr1/RPAP2 lack detectable CTD phosphatase activity We next attempted to demonstrate Pol II CTD pSer5 phosphatase activity with our purified protein samples of His-tagged Rtr1 from K. lactis , A. gossypii , S. cerevisiae and several other fungal species. To test the possibility that Rtr1 in the absence of zinc or in complex with a different metal ion could be catalytically active, we used protein samples purified from E. coli cells that were grown without additional zinc in the medium. The zinc occupancy ranged between 10 and 80%, but other metal ions could be present in these samples. We also expressed and purified residues 1–332 of human RPAP2, as His-tagged and GST-fusion proteins, and full-length RPAP2 as a GST-fusion protein [18] . Despite extensive efforts and using a large collection of different substrates ( Supplementary Table S1 ), we failed to detect CTD pSer5 phosphatase activity for Rtr1 and RPAP2 under any of the conditions tested, while robust activity was observed with Ssu72. The substrates used include a CTD peptide Ser7′′-Tyr1-Ser2-Pro3-Thr4-Ser5-Pro6-Ser7-Tyr1′-Ser2′ phosphorylated at the Ser5, Ser5 and Ser7, or Ser2, Ser5 and Ser7 positions, as it has been shown that RPAP2 requires Ser7 phosphorylation to interact with the CTD [18] . These assays monitored the release of free phosphate from the reactions. We also used as the substrate the entire CTD purified as a GST-fusion protein [10] and either phosphorylated with HeLa cell nuclear extract or purified Cdk7. The reactions were monitored by western blotting with an antibody specific for pSer5. We again failed to detect activity with multiple Rtr1/RPAP2 samples and under a variety of conditions ( Fig. 3a and b and results not shown). In addition, we soaked Rtr1 crystals with CTD phosphopeptides, but were not able to identify any binding based on the crystallographic analysis. 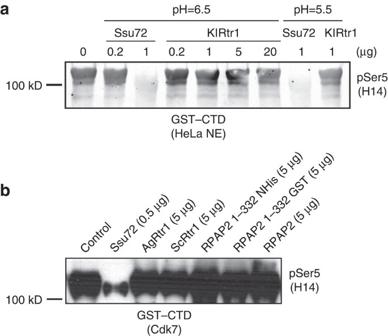Figure 3: Rtr1 and RPAP2 failed to show phosphatase activity with GST–CTD as the substrate. (a) With the GST–CTD substrate phosphorylated by HeLa cell nuclear extract, KlRtr1 shows no signs of activity under various conditions. (b) Phosphatase activity of Rtr1 from different species and human RPAP2 was tested against GST–CTD substrate phosphorylated by the Cdk7 complex. Ssu72 was used as a positive control in both cases. Figure 3: Rtr1 and RPAP2 failed to show phosphatase activity with GST–CTD as the substrate. ( a ) With the GST–CTD substrate phosphorylated by HeLa cell nuclear extract, KlRtr1 shows no signs of activity under various conditions. ( b ) Phosphatase activity of Rtr1 from different species and human RPAP2 was tested against GST–CTD substrate phosphorylated by the Cdk7 complex. Ssu72 was used as a positive control in both cases. Full size image The structure of Rtr1 lacks an apparent active site The lack of phosphatase activity for Rtr1 is consistent with our structure, which does not indicate the presence of an active site. An analysis of the surface features that are conserved among Rtr1 and RPAP2 homologues does not reveal any pockets that are lined with conserved residues and could function as an active site ( Fig. 4 ). The C-terminal segment that is missing in the current structure is unlikely to form an active site, owing to its poor conservation ( Fig. 1 ). The zinc-binding site cannot be an active site either, as the zinc ion is tetrahedrally coordinated by the four ligands and is not capable of binding and activating a water molecule for hydrolytic activity. Moreover, the zinc-binding site corresponds to a small protrusion on the surface of Rtr1 ( Fig. 4 ), and there is no pocket nearby that could bind the CTD substrate. Mutation of one of the Zn ligands in ScRtr1 (Cys73) was reported to abolish the dephosphorylation of pSer5 in yeast cells [16] . It is more likely that this mutation disrupted zinc binding and thereby the overall structure of the protein. We do not know why phosphatase activity was observed in vitro in the earlier reports [16] , [18] . A co-purifying protein with this activity might be a possibility. Figure 4: The structure of Rtr1 does not show evidence for an active site. Molecular surface of K. lactis Rtr1 (front and back views), coloured based on sequence conservation [36] , from highly conserved (purple) to poorly conserved (blue) residues. The highly conserved surface patches are labelled. Full size image If Rtr1/RPAP2 is not a phosphatase, what then is its function in Pol II transcription? Rtr1 is found primarily in the cytoplasm, but can shuttle into the nucleus [15] . Recent reports suggest that Rtr1 and RPAP2 may have an important role in the assembly and transport of Pol II from the cytoplasm into the nucleus [24] , [25] , [26] . These and other [15] , [16] , [17] , [18] data establish that Rtr1 interacts with Pol II, and therefore it is likely that Rtr1 could mediate interactions among various proteins in the Pol II complex. Given the evidence that Rtr1/RPAP2 is important for pSer5 dephosphorylation in vivo [16] , [18] , an attractive possibility is that Rtr1/RPAP2 is required for recruitment and/or activation of the actual phosphatase that dephosphorylates pSer5 during the early stages of Pol II transcription. The identity of that phosphatase remains to be determined. Protein expression and purification Full-length Rtr1 from K. lactis , A. gossypii , S. cerevisiae and the N-terminal region (residues 1–332) of human RPAP2 were cloned into the pET28a vector (Novagen) and overexpressed in E. coli BL21 (DE3) Star cells at 20 °C by the addition of 0.5 mM isopropyl-β- D -thiogalactopyranoside at OD 600 of 0.6. To help the zinc enrichment in the protein, 0.1 mM ZnSO 4 was added to the culture 1 h before induction. The expression constructs introduced hexa-histidine tags at the N terminus of the proteins. The soluble proteins were purified by Ni-NTA (Qiagen) with the elution buffer containing 20 mM Tris (pH 7.5), 200 mM NaCl and 250 mM imidazole, followed by gel filtration (Sephacryl S-300, GE Healthcare) chromatography in a running buffer of 20 mM Tris (pH 7.5), 200 mM NaCl and 2 mM DTT. The proteins were concentrated to 20 mg ml −1 in a buffer containing 20 mM Tris (pH 7.5), 200 mM NaCl, 2 mM DTT and 5% (v/v) glycerol, flash frozen in liquid nitrogen and stored at −80 °C. The GST fusion RPAP2 proteins were made by cloning the full-length human RPAP2 or the N-terminal region (residues 1–332) into pGEX-4T-3 (GE Life Sciences) vector and overexpressed in E. coli BL21 (DE3) Star cells with the same protocol as mentioned above. The proteins were purified by glutathione Sepharose 4 Fast Flow (GE Healthcare) with 20 mM reduced glutathione in a buffer of 20 mM Tris (pH 7.5), 200 mM NaCl and 5% (v/v) glycerol. Protein crystallization Crystals of KlRtr1 were obtained with the sitting-drop vapour diffusion method at 20 °C. The reservoir solution contained 100 mM CHES (pH 9.5) and 20% (w/v) PEG8000. The crystals belong to space group P 2 1 2 1 2 1 , and there are two molecules in the asymmetric unit. Crystals of AgRtr1 were obtained with the sitting-drop vapour diffusion method at 20 °C. The reservoir contained 120 mM Tris (pH 7.0) and 16% (v/v) ethanol. The crystals belong to space group I 422, and there is one molecule in the asymmetric unit. The crystals were cryo-protected by the respective reservoir solutions supplemented with 25% (v/v) ethylene glycol and flash frozen in liquid nitrogen for data collection at 100 K. Data collection and structure determination X-ray diffraction data were collected on an ADSC charge-coupled device at the X29A beamline of National Synchrotron Light Source (NSLS). The diffraction images were processed and scaled with the HKL package [27] . The atomic coordinates of the KlRtr1 structure have been deposited in the Protein Data Bank under the accession code 4FC8 . Multiple-wavelength anomalous diffraction data sets were collected on the KlRtr1 crystal to 2.5 Å resolution, at the zinc absorption edge (inflection point, 1.2836 Å), peak (1.2833 Å) and remote (1.2652 Å) wavelengths. The data processing statistics are summarized in Table 1 . The Zn sites were located with the program BnP [28] . Reflection phases were calculated using the program SOLVE/RESOLVE [29] . The complete atomic model was fit into the electron density with the programs O [30] and Coot [31] . The structure refinement was carried out with the programs CNS [32] and Refmac [33] , against the data set at the peak wavelength. The statistics on the structure refinement are summarized in Table 1 . For the final atomic model, 95.2% of the residues are in the most favoured region of the Ramachandran plot, 4.8% in additional allowed regions and none in the disallowed region. For the AgRtr1 crystal, a single-wavelength anomalous diffraction data set to 3.5 Å resolution was collected at the zinc peak wavelength. An electron density map was obtained based on the single-wavelength anomalous diffraction data, which showed clear indications for several helices. The atomic model of KlRtr1 could be readily positioned into the density, revealing an extra helix in the C-terminal region in the AgRtr1 structure. Refinement of this structure model was not carried out due to the limited resolution. CTD peptide phosphatase assays Reaction mixtures (25 μl) in the standard phosphatase condition (50 mM Bis-Tris (pH 6.5), 20 mM KCl, 10 mM MgCl 2 and 5 mM DTT) containing 500 μM CTD peptide, Rtr1, RPAP2 or Ssu72 at 1 μM, 5 μM or 20 μM concentration were incubated at 30 °C. Time-point samples were taken and quenched by adding 0.5 ml of malachite green reagent (BIOMOL Research Laboratories, Plymouth Meeting, PA). Phosphate release was determined by measuring A 620 and comparing it with a phosphate standard curve. CTD phosphatase assay Purified GST–CTD fusion protein was phosphorylated in vitro by HeLa cell nuclear extract as described [34] , or by Cdk7 complex as described [35] . CTD phosphatase assays were performed in a total volume of 20 μl in the standard phosphatase condition containing 200 ng phosphorylated GST–CTD and indicated amount of Rtr1, RPAP2 or Ssu72. Reactions were incubated for 1 h at 30 °C, stopped by adding 5 μl 5× SDS loading buffer and 2.5 μl from each reaction was resolved on an 8% SDS–PAGE gel. pSer5 level was detected by western blot using H14 antibody (Covance). All CTD peptide phosphatase assays and CTD phosphatase assays were additionally performed in different conditions by varying pH (5.5–8.5) or KCl concentration (20–500 mM) or additives (1–10 mM ZnCl 2 or MnCl 2 or MgCl 2 ) based on the standard phosphatase condition. Accession codes: The atomic coordinates of the KlRtr1 structure have been deposited in the Protein Data Bank under the accession code 4FC8 . How to cite this article: Xiang, K. et al . The yeast regulator of transcription protein Rtr1 lacks an active site and phosphatase activity. Nat. Commun. 3:946 doi: 10.1038/ncomms1947 (2012).